Multi-peaked adaptive landscape for chikungunya virus evolution predicts continued fitness optimization inAedes albopictus mosquitoes Host species-specific fitness landscapes largely determine the outcome of host switching during pathogen emergence. Using chikungunya virus (CHIKV) to study adaptation to a mosquito vector, we evaluated mutations associated with recently evolved sub-lineages. Multiple Aedes albopictu s-adaptive fitness peaks became available after CHIKV acquired an initial adaptive (E1-A226V) substitution, permitting rapid lineage diversification observed in nature. All second-step mutations involved replacements by glutamine or glutamic acid of E2 glycoprotein amino acids in the acid-sensitive region, providing a framework to anticipate additional A. albopictus -adaptive mutations. The combination of second-step adaptive mutations into a single, ‘super-adaptive’ fitness peak also predicted the future emergence of CHIKV strains with even greater transmission efficiency in some current regions of endemic circulation, followed by their likely global spread. A critical factor determining a pathogen’s potential to emerge and successfully sustain its circulation in new environments to cause new disease is its ability to undergo genetic adaptation to new recipient hosts. The number and nature of host-switching adaptations for a given pathogen are largely determined by the shape of the corresponding viral fitness landscapes [1] , [2] , [3] . As highlighted by a recent study of experimental adaptation of highly pathogenic avian H5N1 influenza A viruses for transmission between mammals, detailed information about the shape of adaptive landscapes would allow for targeted assessment of the epidemic potential of a given pathogen strain. This information could provide health authorities with a head start in their efforts to mitigate or prevent the public health impacts of new emergences [4] . However, to our knowledge, no detailed characterization of the adaptive landscapes exists for any important pathogen, primarily owing to the complexity of experimental settings and conditions needed to accurately recreate in the laboratory the conditions required for natural transmission and maintenance. To overcome this limitation, we utilized a combination of phylogenetic and experimental approaches to study recent events in chikungunya virus (CHIKV) evolution that will facilitate the inference of future emergence trends. A novel lineage of the mosquito-borne CHIKV ( Togaviridae : Alphavirus ) emerged in 2004 in coastal Kenya, followed by its expansive spread via infected travellers to produce a series of epidemics of severe, often chronic arthralgic disease throughout the Indian Ocean basin and Southeast Asia, as well as in Europe ( Fig. 1a ) [5] , [6] . It has been estimated that these emerging CHIKV strains from the Indian Ocean lineage (IOL) have infected up to 10 million people to cause debilitating arthralgia [5] , [6] and have also been implicated in several thousand human deaths [7] , [8] , [9] . Unlike previous epidemics, where CHIKV was transmitted among humans primarily by the highly urbanized, tropical mosquito Aedes ( Stegomyia ) aegypti , A. ( Stegomyia ) albopictus has been incriminated as the primary CHIKV vector during the majority of recent IOL outbreaks, including those on several islands of the western Indian Ocean, parts of India, Singapore, Malaysia, Thailand, Sri Lanka, China and Italy [10] , [11] , [12] , [13] , [14] , [15] . This highly invasive mosquito has spread since 1985 from its native distribution in Asia to all continents except Antarctica [16] . Furthermore, unlike A. aegypti , A. albopictus survives in both tropical and temperate climates, permitting it to transmit CHIKV in northern latitudes such as Italy [17] . 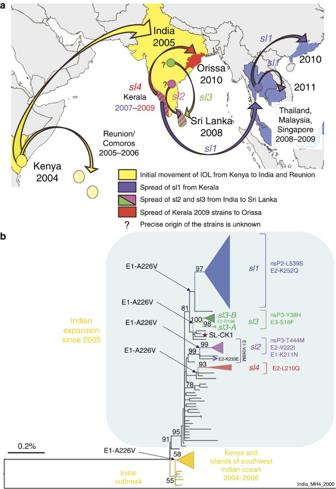Figure 1: Phylogenetic relationships and spread of IOL CHIKV strains in the Indian Ocean region since 2004. (a) Origin and reconstructed spread of sl1-3 and Kerala 2009 (sl4) strains. (b) Phylogenetic tree generated using complete genomic sequences of 91 representative IOL CHIKV strains constructed using the maximum likelihood method. Bootstrap values, sl1-4-specific and E1-A226V mutations are indicated. The SL07 strain used as a genetic background for allin vivoexperiments is highlighted with an asterisk. The purple arrow highlights strain LK(EH)CH18608 with the E2-K233E substitution. The bar indicates 0.2% nucleotide sequence divergence. Figure 1: Phylogenetic relationships and spread of IOL CHIKV strains in the Indian Ocean region since 2004. ( a ) Origin and reconstructed spread of sl1-3 and Kerala 2009 (sl4) strains. ( b ) Phylogenetic tree generated using complete genomic sequences of 91 representative IOL CHIKV strains constructed using the maximum likelihood method. Bootstrap values, sl1-4-specific and E1-A226V mutations are indicated. The SL07 strain used as a genetic background for all in vivo experiments is highlighted with an asterisk. The purple arrow highlights strain LK(EH)CH18608 with the E2-K233E substitution. The bar indicates 0.2% nucleotide sequence divergence. Full size image A. albopictus- adaptive mutations in the E1 and E2 envelope glycoproteins (E1-A226V and E2-L210Q, respectively) in emerging IOL strains are believed to have played critical roles in the unprecedented scale of the ongoing epidemic [18] . The E1-A226V substitution provided a major fitness increase (50–100-fold) [19] followed by an additional fitness increase (four to sixfold), caused by E2-L210Q, once CHIKV reached the initial A. albopictus -adaptive fitness peak [18] . This stepwise adaptive process for this cross-species arbovirus jump [18] , [20] was similar to the adaptive emergence of the SARS coronavirus for human-to-human transmission [21] . Phylogenetic and epidemiologic studies indicate that E1-A226V was selected convergently by at least four different CHIKV lineages in different geographic locations [6] , [11] , [12] , [14] , [22] , [23] , [24] , whereas E2-L210Q was detected only in closely related strains from states of Kerala and Orissa, India in 2009 and 2010, respectively [25] , [26] ( Fig. 1a ). Interestingly, E2-210Q is absent in all other CHIKV sub-lineages that acquired the E1-A226V change ( Fig. 1b ), posing the question of whether acquisition of this second-step A. albopictu s-adaptive substitution was a unique event in CHIKV evolution, or whether other viral sub-lineages have acquired different second-step mutations (to occupy independent A. albopictus -adaptive peaks), which like the effect of E2-L210Q, further increase CHIKV fitness for infection of A. albopictu s. To address this question, we performed a comprehensive investigation of mutations associated with recently evolved CHIKV sub-lineages and their possible effects on viral fitness. Several sub-lineage-specific, second-step A. albopictus -adaptive mutations were identified, all involving replacements by glutamine or glutamic acid in the acid-sensitive region (ASR) of the E2 glycoprotein. These findings indicate that, after acquisition of an initial A. albopictus -adaptive (E1-A226V) substitution, multiple second-step fitness peaks became available for CHIKV, enabling rapid lineage diversification. Apparent structural and functional similarities observed among all second-step A. albopictus -adaptive mutations enabled predictions of additional A. albopictus -adaptive CHIKV mutations. Finally, analysis of CHIKV expressing a combination of second-step adaptive mutations revealed the existence of a ‘super- A. albopictus -adaptive’ fitness peak, which suggested the future emergence of CHIKV strains with even greater transmission efficiency in the future. Fitness of CHIKV sub-lineages 1, 2 and 3 Comprehensive phylogenetic analyses of CHIKV strains within the IOL identified that, in addition to the 2009 Kerala sub-lineage ( sl ) associated with the E2-L210Q second-step A. albopictu s-adaptive substitution, three additional CHIKV sl s included E1-226 V, each with a unique genetic signature ( Fig. 1b ). A detailed phylogenetic tree containing name of strains and year and location of isolation is available in Supplementary Fig. 1 ) [11] . Viruses from sl1 included two novel mutations encoding nsP2-L539S and E2-K252Q, which were first detected in Kerala, India in 2007 (2 years before the appearance of E2-L210Q). This sl1 subsequently spread into Southeast Asia, where it was isolated beginning in 2008. The last isolates were reported in 2012 in Cambodia [27] , suggesting its persistence in the region. Viruses from sl2 and sl3 were identified only in 2008 during a Sri Lankan outbreak and have not been reported since [11] . The genetic signature of sl2 consisted of four novel substitutions (nsP3-T444M, E2-V222I, E1-K211N and E1-V269M), with E1-V269M predicted phylogenetically to have occurred before the E1-A226V substitution. Strains of sl3 acquired two novel substitutions (nsP3-Y38H and E3-S18F) ( Fig. 1b ; Supplementary Fig. 1 ). Because the sl from Kerala, 2009 appeared most recently, we refer to it as sl4 . To determine whether any of the additional mutations in sl1-3 produce second-step A. albopictu s-adaptive substitutions, the nonsynonymous mutations described above were introduced into the SL07-226V_Apa CHIKV strain, which was generated based on the SL-CK1 strain isolated in 2007 in Sri Lanka ( Fig. 1b , asterisk) [18] . The complementary DNA (cDNA) clone used to generate this strain was genetically marked with a synonymous mutation that ablated an Apa I restriction site, allowing for the determination of its ratio to competitors by reverse transcriptase (RT)-PCR followed by a restriction digest of amplicon DNA. Changes in this ratio before and after competition infections indicated relative fitness values of the mutant compared with the SL07-226V_Apa CHIKV strain. Viruses were rescued by RNA electroporation into Vero cells and fitness for A. albopictu s infection of SL07-226V_Apa was assessed in direct competition experiments against the unmarked, wild-type (wt) SL07-226V strain; the synonymous marker itself does not affect CHIKV fitness in vitro or in vivo [19] . Infections that disseminated from the mosquito midgut into the haemocoel, a requirement for transmission, were assessed by detection of CHIKV in the head, while initial infection was determined by detection of virus in the remainder of the mosquito body. Both SL07-226V_Apa and SL07-226V viruses contained the first-step E1-A226V-adaptive substitution, representing a typical genetic background of IOL strains from India upon which selection of second-step mutations occurred. In addition to sequencing each cDNA clone to ensure that no errors accompanied mutagenesis, the genetic integrity of mutagenized viruses was ensured by comparison of the specific infectivity of viral RNA and virus titres post electroporation into Vero cells ( Supplementary Tables 1–5 ). Introduction of the double mutation (nsP2-L539S/E2-K252Q) from sl1 into the SL07-226V_Apa backbone ( Fig. 2a ) resulted in a virus that was significantly more efficient in developing a disseminated infection in A. albopictu s, as measured by mosquito head infections (one-tailed McNemar test P =0.011), compared with SL07-226V ( Fig. 2b ). In addition, these combined nsP2-L539S/E2-K252Q substitutions resulted in a mean 7.8-fold increase in the SL07-226V_Apa- sl1 :SL07-226V RNA ratio in A. albopictus bodies ( Fig. 2d ) assayed 10 days post infection (dpi). To validate these results, we repeated our analysis using a different, uncloned, natural sl1 virus strain, Thailand-2009_CK11/53, isolated from a febrile patient ( Supplementary Fig. 1 ), which also contained the signature sl1 nsP2-L539S/E2-K252Q substitutions. This virus was competed against the clone-derived SL07-226V_Apa strain in A. albopictus mosquitoes from a Thai colony. Similar to the SL07-226V_Apa- sl1 virus, Thailand-2009_CK11/53 was 5.8-fold more efficient in developing a disseminated mosquito infection compared with SL07-226V_Apa (one-tailed McNemar test, P =0.0001), and also outcompeted SL07-226V_Apa in bodies of A. albopictus assayed 10 dpi ( Supplementary Fig. 2 ). These data confirmed that sl1 CHIKV strains acquired second-step mutations other than E2-L210Q to increase their fitness for A. albopictus infection. 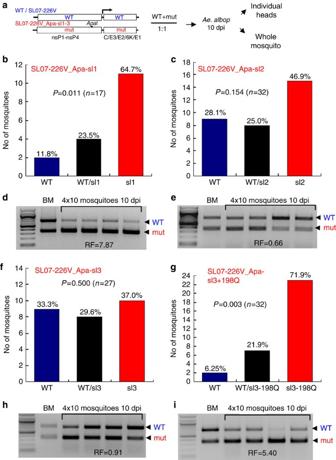Figure 2: Effect of sl1-3-specific mutations on CHIKV fitness following competition inA. albopictus. (a) Schematic representation of the experimental design.A. albopictusmosquitoes from a Thai colony were presented with blood meals (BM) containing 106p.f.u. ml−1of a 1:1 mixture of viruses (based on p.f.u.) expressing either sl1 (b,d), sl2 (c,e), sl3 (f,h) or sl3-B (g,i) signature mutations and wt (SL07-226) virus, and processed at 10 dpi. Graphs (b,c,f,g) show numbers and percentages of mosquitoes containing mutant (mut), wt or both viruses in individual mosquito heads (representing disseminated infections). For each virus pair, the difference in number of mosquitoes with disseminated infection of mutant versus wt was tested for significance with a one-tailed McNemar test. Gel images (d,e,h,i) show change in relative RNA levels for each virus competition pair. RNA was extracted from BM at 0 dpi or 4 pools of 10 mosquitoes per pool at 10 dpi followed by RT-PCR analysis andApaI digestion to distinguish marked from unmarked competitors. The relative fitness (RF) was determined as a geometric mean of the ratio between mut:wt bands in the sample amplicon, divided by the starting ratio of mut:wt bands in the BM amplicon. Figure 2: Effect of sl1-3-specific mutations on CHIKV fitness following competition in A. albopictus. ( a ) Schematic representation of the experimental design. A. albopictus mosquitoes from a Thai colony were presented with blood meals (BM) containing 10 6 p.f.u. ml −1 of a 1:1 mixture of viruses (based on p.f.u.) expressing either sl1 ( b , d ), sl2 ( c , e ), sl3 ( f , h ) or sl3-B ( g , i ) signature mutations and wt (SL07-226) virus, and processed at 10 dpi. Graphs ( b , c , f , g ) show numbers and percentages of mosquitoes containing mutant (mut), wt or both viruses in individual mosquito heads (representing disseminated infections). For each virus pair, the difference in number of mosquitoes with disseminated infection of mutant versus wt was tested for significance with a one-tailed McNemar test. Gel images ( d , e , h , i ) show change in relative RNA levels for each virus competition pair. RNA was extracted from BM at 0 dpi or 4 pools of 10 mosquitoes per pool at 10 dpi followed by RT-PCR analysis and Apa I digestion to distinguish marked from unmarked competitors. The relative fitness (RF) was determined as a geometric mean of the ratio between mut:wt bands in the sample amplicon, divided by the starting ratio of mut:wt bands in the BM amplicon. Full size image The combined expression of all signature sl2 nonsynonymous mutations (nsP3-T444M/E2-V222I/E1-K211N/E1-V269M) in the SL07-226V_Apa genome did not significantly affect CHIKV’s ability to develop a disseminated infection in A. albopictu s ( Fig. 2c , one-tailed McNemar test, P =0.154), nor did it result in an apparent change in the ratio of SL07-226V_Apa- sl2 versus SL07-226V RNA in mosquito bodies at 10 dpi ( Fig. 2e ). Similarly, the individual expression of each of these sl2 substitutions in the SL07-226V background did not significantly affect its ability to develop a disseminated infection ( Supplementary Fig. 3 ; one-tailed McNemar test, P >0.05). Additional analysis of the structural gene sequences of sl2 strains did not reveal any other novel mutations shared by >2 strains for which genomic sequences were available in GenBank. On the basis of these data, we concluded that sl2 did not evolve second-step A. albopictu s-adaptive mutations. Introduction of nonsynonymous signature mutations from sl3 (nsP3-Y38H/E3-S18F) into SL07-226V_Apa did not significantly affect its ability to develop a disseminated infection in A. albopictu s ( Fig. 2f,h ; one-tailed McNemar test, P =0.5). However, a dn/ds analysis of sl3 sequences revealed a novel, putative positively selected E2-R198Q substitution ( Supplementary Table 6 ), which was present only in strains of clade sl3-B , but not in sl3-A ( Fig. 1b ). Position E2-198 mapped to a region adjacent to E2-210 in the crystal structure of the CHIKV E2 protein [28] , suggesting that like E2-L210Q, E2-R198Q affects CHIKV infection of A. albopictus . 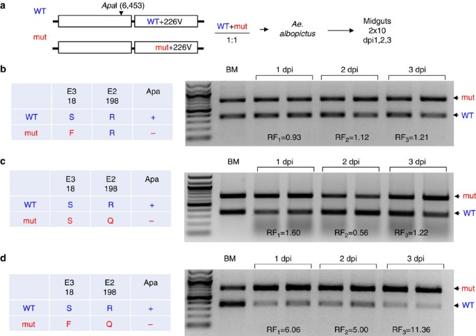Figure 6: Effect of individual or combined expression of sl3-B-specific mutations on CHIKV initial infection and replication in midguts ofA. albopictus. (a) Schematic representation of the experimental design. A 1:1 ratio (based on p.f.u.) of viruses that differ by the sets of indicated substitutions (see tables on the left of each figure) was presented to a Thailand colony ofA. albopictusat final blood meals (BM) titre of 1 × 106p.f.u. ml−1. At 1, 2 and 3 dpi, mosquito midguts were collected in pools of 10. RNA was extracted from each pool followed by RT-PCR analysis andApaI digestion. (b–d) Tables show genetic differences between the competing viruses. The relative fitness (RF) for each time point was determined as the geometric mean of the ratio of mut to wt bands in amplicons derived from each sample, divided by the starting ratio of mut and wt bands in the BM amplicon. Introduction of E2-R198Q into the SL07-226V_Apa- sl3 backbone resulted in a virus that was 11.5-fold more efficient in developing a disseminated infection in A. albopictu s ( Fig. 2g ; one-tailed McNemar test, P =0.003), and that increased by 5.4-fold the ratio of its RNA in mosquito bodies relative to SL07-226V at 10 dpi ( Fig. 2i ). These data indicated that, like sl1 , the Sri Lankan CHIKV sl3-B independently acquired a second-step mutation other than E2-L210Q that increased fitness for infection of A. albopictus. To investigate whether signature substitutions from sl1 (nsP2-L539S/E2-K252Q) and from sl3-B (nsP3-Y38H/E3-S18F/E2-R198Q; corresponds to sl3+198Q ) were selected specifically by A. albopictu s, we compared their effects on CHIKV fitness in the other main epidemic mosquito vector, A. aegypti. We also assessed fitness in Vero African green monkey kidney and human foreskin fibroblast (HFF) cell lines (fibroblasts are considered to be initial sites of human infections) [29] , and in a surrogate human model, 2-day-old infant mice, using competition assays against SL07-226V. Although they had no effect on fitness for A. albopictus , the sl2 mutations were also included in these experiments. The sl1 , sl2 and sl3-B mutations had no significant effect on dissemination of CHIKV into the heads of A. aegypti (one-tailed McNemar test, P >0.05). In addition, there was no increase in the relative RNA ratio associated with mutations from sl1 , sl2 and sl3-B versus SL07-226V in A. aegypti bodies at 10 dpi ( Supplementary Fig. 4 ), indicating that these mutations did not increase CHIKV fitness for infection of this vector. Similarly, the relative RNA SL07-226V_Apa- sl1 :SL07-226V_Apa- sl3-B ratio was not increased in supernatants of Vero and HFF cells over SL07-226V, when assayed at 1 and 2 dpi ( Fig. 3 ). Infection of 2-day-old mice with mixtures of SL07-226V and SL07-226V_Apa- sl1 or SL07-226V_Apa- sl3-B led to slight decreases in the relative RNA amount of the latter strain at 1 dpi in mouse blood, which subsequently increased to equal amounts at 2 dpi ( Fig. 4 ). These data suggest the lack of an overall fitness gain in these surrogate CHIKV human models associated with mutations from sl1 and sl3-B, supporting the hypothesis that some if not all of these mutations were selected specifically by A. albopictus . Interestingly, only SL07-226V_Apa- sl2 exhibited increased fitness over SL07-226V in infant mice at a single time point (1 dpi; Fig. 4c ). This might indicate that at least some sl2 mutations were acquired as a result of CHIKV adaptation to a vertebrate host, presumably humans. 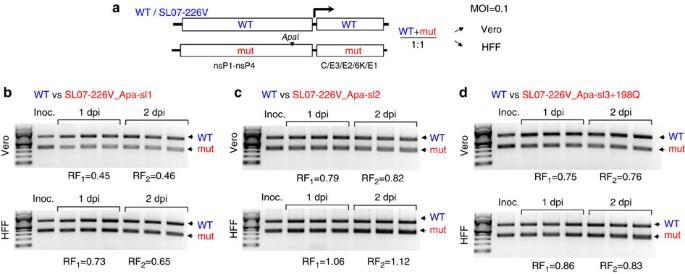The restoration of the viral competitors’ ratio to almost 1:1 in the serum of all of mice analysed on 2 dpi suggests that their replication occurred independently from one another, and that they reached plateaus at different times, rather than accumulation of additional mutations affecting the competition outcome. Figure 3: Effect of sl1, sl2 and sl3-B-specific mutations on CHIKV fitness in Vero and HFF cells. (a) Schematic representation of the experimental design. Cells were infected at a multiplicity of 0.1 p.f.u. per cell in triplicate with a 1:1 mixture of viruses (based on p.f.u.) expressing either sl1- (b), sl2- (c) or sl3-B-specific (d) mutations (mut) and SL07-226V (wt) virus. At 1 and 2 dpi, supernatants were collected for RNA extraction and RT-PCR analysis. The relative fitness (RF) within a given competition was determined as the geometric mean of the ratio between mut and wt bands in the sample amplicon, divided by the starting ratio of mut to wt bands in the amplicon derived from the inoculum used for infection of cells. Figure 3: Effect of sl1, sl2 and sl3-B-specific mutations on CHIKV fitness in Vero and HFF cells. ( a ) Schematic representation of the experimental design. Cells were infected at a multiplicity of 0.1 p.f.u. per cell in triplicate with a 1:1 mixture of viruses (based on p.f.u.) expressing either sl1- ( b ), sl2- ( c ) or sl3-B-specific ( d ) mutations (mut) and SL07-226V (wt) virus. At 1 and 2 dpi, supernatants were collected for RNA extraction and RT-PCR analysis. 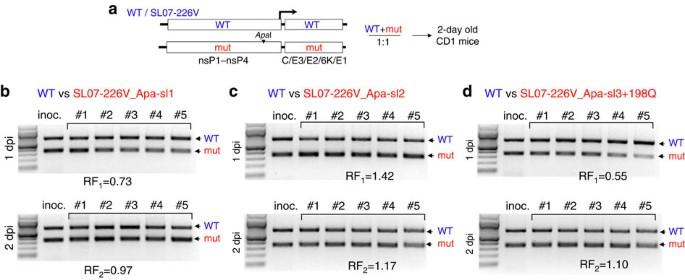The relative fitness (RF) within a given competition was determined as the geometric mean of the ratio between mut and wt bands in the sample amplicon, divided by the starting ratio of mut to wt bands in the amplicon derived from the inoculum used for infection of cells. Figure 4: Effect of sl1-, sl2- and sl3-B-specific mutations on CHIKV fitness in infant mice. (a) Schematic representation of the experimental design. 2 to 3-day-old CD-1 mice were infected with 102p.f.u. of a 1:1 mixture of viruses (based on p.f.u.) expressing sl1- (b), sl2- (c) or sl3-B-specific (d) mutations (mut) and SL07-226V (wt) virus. At 1 and 2 dpi, CHIKV RNA was extracted from the blood of individual mice and used for RT-PCR analysis. The relative fitness (RF) within a given competition was determined as the geometric mean of the ratio of mut to wt bands in amplicons derived from the mouse blood, divided by the starting ratio of mut and wt bands in the amplicon from the inoculum used for infection of mice. Full size image Figure 4: Effect of sl1-, sl2- and sl3-B-specific mutations on CHIKV fitness in infant mice. ( a ) Schematic representation of the experimental design. 2 to 3-day-old CD-1 mice were infected with 10 2 p.f.u. of a 1:1 mixture of viruses (based on p.f.u.) expressing sl1- ( b ), sl2- ( c ) or sl3-B-specific ( d ) mutations (mut) and SL07-226V (wt) virus. At 1 and 2 dpi, CHIKV RNA was extracted from the blood of individual mice and used for RT-PCR analysis. The relative fitness (RF) within a given competition was determined as the geometric mean of the ratio of mut to wt bands in amplicons derived from the mouse blood, divided by the starting ratio of mut and wt bands in the amplicon from the inoculum used for infection of mice. Full size image To evaluate which specific mutations in sl1 and sl3-B influence CHIKV fitness in A. albopictus , (nsP2-L539S/E2-K252Q) from sl1 and (nsP3-Y38H/E3-S18F/E2-R198Q) from sl3-B were introduced individually or in combinations into SL07-226V, and the resultant viruses were tested in competition assays against SL07-226V_Apa using A. albopictus . The E2-K252Q substitution caused a significant increase in the ability of CHIKV to develop a disseminated infection (one-tailed McNemar test, P ≤0.001), and resulted in a >5.9-fold increase in the relative RNA ratio over SL07-226V_Apa in bodies of mosquitoes from Thailand and Galveston colonies ( Supplementary Fig. 5a ). Introduction of nsP2-L539S into SL07-226V also resulted in a slight but insignificant fitness increase in the level of CHIKV dissemination (one-tailed McNemar test, P =0.076) and relative RNA ratio versus SL07-226V in both colonies of A. albopictu s ( Supplementary Fig. 5b ). However the fitness of SL07-226V_Apa expressing nsP2-L539S and E2-K252Q was indistinguishable (one-tailed McNemar test, P =0.5) from SL07-226V expressing only the single E2-K252Q substitution ( Supplementary Fig. 5c ), indicating that only E2-K252Q and not nsP2-L539S plays a major role in the fitness increase of sl1 strains for infection of A. albopictu s. Surprisingly, the individual expression of sl3-B substitutions nsP3-Y38H, E3-S18F and E2-R198Q in the SL07-226V backbone had no significant effect (one-tailed McNemar test, P >0.05) on the ability of CHIKV to develop a disseminated infection in A. albopictu s from Thailand ( Supplementary Fig. 6b–d ). These results suggested that some of these mutations could be influenced by epistatic interactions. Indeed, simultaneous expression of only the E3-S18F and E2-R198Q substitutions in SL07-226V generated a 11.5-fold increase in the ability to develop a disseminated infection in A. albopictu s (one-tailed McNemar test, P <0.001) and resulted in a 10.2-fold increase in the relative RNA amount in mosquito bodies over SL07-226V ( Supplementary Fig. 6e ), to the level previously observed for the triple mutant SL07-226V_Apa- sl3+198Q ( Fig. 2g,i ). These results indicated that, for sl3-B , second-step adaptation to A. albopictu s was achieved by the acquisition of two synergistic mutations, E3-S18F and E2-R198Q. Considering that E2-R198Q was selected in the sl3 background, which had already acquired E3-S18F ( Fig. 1b ), the acquisition of E2-R198Q was likely the result of direct selection by A. albopictu s. The evolutionary basis of the E3-S18F substitution in sl3 remains unknown, but it may have resulted from a founder effect or drift if it confers no phenotype on its own. Mutations act through common adaptive mechanism An intriguing common feature of novel A. albopictu s-adaptive mutations from sl1 and sl3-B is that they all result in the acquisition of glutamine residues in the E2 glycoprotein (E2-252Q and E2-198Q), like the A. albopictu s-adaptive E2-L210Q substitution previously characterized in sl4 [18] . As described above, CHIKV fitness for A. albopictus infection was not significantly affected by the sl2 mutations, which may reflect that this sl was the only one that did not acquire glutamine E2 substitutions ( Fig. 2c,e ; Supplementary Fig. 3 ). Previously, we demonstrated that E2-L210Q primarily mediates more efficient initial CHIKV infection of A. albopictu s midgut cells, which subsequently leads to more efficient dissemination into the haemocoel [18] . To investigate whether the similarities among the E2-252Q, E2-198Q and E2-210Q substitutions reflect a common effector mechanism, we analysed the impact of these substitutions on CHIKV fitness during initial infection/replication of/in the A. albopictus midgut. The E2-L252Q mutation alone and combined (E3-S18F/E2-R198Q) mutations were responsible for 5.7- and 6.1-fold increases in the relative CHIKV RNA ratios, respectively, over control SL07-226V_Apa, as early as 1 dpi ( Figs 5 and 6 ). These results support the hypothesis of a common effector mechanism for all second-step A. albopictu s-adaptive mutations. Interestingly, the E2-R198Q sl3-B substitution alone was also associated with a small (1.6-fold) increase in its RNA ratio in mosquito midguts at 1 dpi, but this effect did not extend to day 2, when SL07-226V_Apa rebounded ( Fig. 6c ). 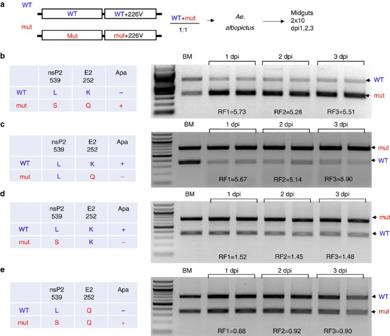More rapid replication of SL07-226V_Apa between 1 and 2 dpi might be explained if E2-R198Q promotes initial CHIKV infectivity of midgut cells, while E3-S18F stabilizes (probably via an indirect interaction) the E2 glycoprotein with 198Q during spike and virion assembly in midgut cells. Figure 5: Effect of individual or combined expression of sl1–specific mutations on CHIKV initial infection and replication in midguts ofA. albopictus. (a) Schematic representation of the experimental design. A 1:1 ratio (based on p.f.u.) of viruses that differ by the set of indicated substitutions (see tables on the left of each figure) was presented to a Thailand colony ofA. albopictusat a final blood meals (BM) titre of 1 × 106p.f.u. ml−1. At 1, 2 or 3 dpi, mosquito midguts were collected in pools of 10. RNA was extracted from each pool followed by RT-PCR analysis andApaI digestion. (b–e) Tables show genetic differences between the competing viruses. The relative fitness (RF) for each time point was determined as a geometric mean of ratio of mut to wt bands in the amplicon derived from the sample, divided by the starting ratio of mut and wt bands in the BM amplicon. Figure 5: Effect of individual or combined expression of sl1–specific mutations on CHIKV initial infection and replication in midguts of A. albopictus. ( a ) Schematic representation of the experimental design. A 1:1 ratio (based on p.f.u.) of viruses that differ by the set of indicated substitutions (see tables on the left of each figure) was presented to a Thailand colony of A. albopictus at a final blood meals (BM) titre of 1 × 10 6 p.f.u. ml −1 . At 1, 2 or 3 dpi, mosquito midguts were collected in pools of 10. RNA was extracted from each pool followed by RT-PCR analysis and Apa I digestion. ( b – e ) Tables show genetic differences between the competing viruses. The relative fitness (RF) for each time point was determined as a geometric mean of ratio of mut to wt bands in the amplicon derived from the sample, divided by the starting ratio of mut and wt bands in the BM amplicon. Full size image Figure 6: Effect of individual or combined expression of sl3-B-specific mutations on CHIKV initial infection and replication in midguts of A. albopictus. ( a ) Schematic representation of the experimental design. A 1:1 ratio (based on p.f.u.) of viruses that differ by the sets of indicated substitutions (see tables on the left of each figure) was presented to a Thailand colony of A. albopictus at final blood meals (BM) titre of 1 × 10 6 p.f.u. ml −1 . At 1, 2 and 3 dpi, mosquito midguts were collected in pools of 10. RNA was extracted from each pool followed by RT-PCR analysis and Apa I digestion. ( b – d ) Tables show genetic differences between the competing viruses. The relative fitness (RF) for each time point was determined as the geometric mean of the ratio of mut to wt bands in amplicons derived from each sample, divided by the starting ratio of mut and wt bands in the BM amplicon. Full size image E2 mutations lie along a central axis All second-step A. albopictu s-adaptive mutations in the E2 protein shared apparent structural and functional similarities, as well as a spatial arrangement along an axis formed by E2 residues 210–252 ( Fig. 7a ). These similarities raised the hypothesis that the substitution by glutamine of additional amino acids along this E2 axis will also increase fitness for A. albopictu s infection, potentially leading to the selection and emergence of novel CHIKV sub-lineages. To test this hypothesis, we generated five novel CHIKV mutants expressing glutamine along this axis at E2 positions 213, 232, 233, 248 and 254 in the SL07-226V background ( Fig. 7a ) and tested them in competition against SL07-226V_Apa in A. albopictus. These mutations resulted in a range of phenotypes indicated by differences in relative amounts of viral RNA in mosquito bodies and the ability to infect and disseminate into mosquito heads ( Fig. 7 ): (1) slightly attenuated to neutral (E2-T213Q and E2-H232Q, respectively); (2) slightly to moderately beneficial (E2-K254Q and E2-L248Q, respectively); and (3) highly beneficial (E2-K233Q). Introduction of the E2-K233Q substitution into SL07-226V resulted in CHIKV that was fivefold more efficient in developing disseminated A. albopictu s infection (one-tailed McNemar test, P <0.001) and led to a 4.4-fold increase in the relative RNA ratio over the SL07-226V_Apa competitor in mosquito bodies ( Fig. 7k,o ), which closely resembled the phenotypes of A. albopictus- adaptive mutations found in sl1 , sl3-B and sl4 strains ( Fig. 2 ) [18] . This E2-K233Q substitution was also tested for its effect on infection/replication in A. albopictu s midguts during the initial phase of CHIKV infection. A 3.6-fold increase in relative RNA amount was observed in midguts at 1 dpi, which gradually increased to 8.9-fold at 3 dpi ( Supplementary Fig. 7b ). These data suggested that E2-K233Q, similarly to the previously characterized A. albopictu s-adaptive mutations, acts at the levels of initial midgut infection and/or replication. 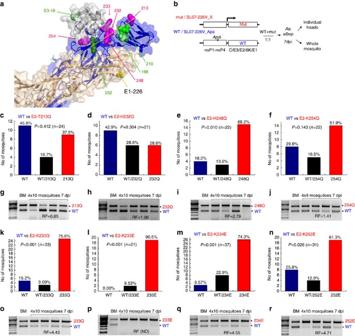Figure 7: Effect of mutations located on E2-210-252 axis on CHIKV fitness inA. albopictus. (a) Atomic structure of the CHIKV E3 (grey)/E2 (blue)/E1 (yellow) spike complex constructed based on (PDB ID:3N4428), demonstrating locations of introduced substitutions (pink spheres). Yellow and green spheres highlight positions of first- and second-step adaptive substitutions. (b) Schematic representation of the experimental design;A. albopictusmosquitoes from a Thai colony were presented with blood meals (BM) containing 106p.f.u. ml−1of a 1:1 mixture of wt (SL07-226V_Apa) and virus containing a single mutation located on E2-210-252 axis (E2-T213Q (c,g), E2-H232Q (d,h), E2-L248Q (e,i), E2-K254Q (f,j), E2-K233Q (k,o), E2-K233E (l,p), E2-K234E (m,q) and E2-K252E (n,r)), and processed at 7 dpi. Graphs (c–f,k–n) show numbers and percent of mosquitoes containing mutant, wt or containing both viruses in individual mosquito heads (representing disseminated infections) as determined from RT-PCR amplicons. For each virus pair the difference in number of mosquitoes with disseminated infection of mutant versus wt was tested for significance with a one-tailed McNemar test. Gel images (g–j,o–r) show change in relative RNA levels for each virus pair. RNA was extracted from BM at 0 dpi or 4 pools of 9–10 mosquitoes per pool at 7 dpi followed by RT-PCR analysis andApaI digestion to distinguish marked (wt) from unmarked (mutant) competitors. The relative fitness (RF) was determined as a geometric mean of the ratio between mut:wt bands in an amplicon derived from the sample, divided by the starting ratio of mut:wt bands in the BM. ND, data not determined. Figure 7: Effect of mutations located on E2-210-252 axis on CHIKV fitness in A. albopictus. ( a ) Atomic structure of the CHIKV E3 (grey)/E2 (blue)/E1 (yellow) spike complex constructed based on (PDB ID:3N44 [28] ), demonstrating locations of introduced substitutions (pink spheres). Yellow and green spheres highlight positions of first- and second-step adaptive substitutions. ( b ) Schematic representation of the experimental design; A. albopictus mosquitoes from a Thai colony were presented with blood meals (BM) containing 10 6 p.f.u. ml −1 of a 1:1 mixture of wt (SL07-226V_Apa) and virus containing a single mutation located on E2-210-252 axis (E2-T213Q ( c , g ), E2-H232Q ( d , h ), E2-L248Q ( e , i ), E2-K254Q ( f , j ), E2-K233Q ( k , o ), E2-K233E ( l , p ), E2-K234E ( m , q ) and E2-K252E ( n , r )), and processed at 7 dpi. Graphs ( c – f,k – n ) show numbers and percent of mosquitoes containing mutant, wt or containing both viruses in individual mosquito heads (representing disseminated infections) as determined from RT-PCR amplicons. For each virus pair the difference in number of mosquitoes with disseminated infection of mutant versus wt was tested for significance with a one-tailed McNemar test. Gel images ( g – j , o – r ) show change in relative RNA levels for each virus pair. RNA was extracted from BM at 0 dpi or 4 pools of 9–10 mosquitoes per pool at 7 dpi followed by RT-PCR analysis and Apa I digestion to distinguish marked (wt) from unmarked (mutant) competitors. The relative fitness (RF) was determined as a geometric mean of the ratio between mut:wt bands in an amplicon derived from the sample, divided by the starting ratio of mut:wt bands in the BM. ND, data not determined. Full size image To explore whether E2-K233Q has been used in nature by CHIKV as an alternative mode of adaptation to A. albopictus , we searched for this mutation in the Genbank library. Although no sequences had E2-233Q, we found E2-233E in one CHIKV isolate that was most closely related to sl2 , the only sub-lineage for which we did not find A. albopictus -adaptive mutations in signature sequences ( Fig. 1b ). Interestingly, the same residue was found previously in a CHIKV antibody escape mutant that had been passaged in A. albopictus -derived C6/36 cells, but not in baby hamster kidney (BHK-21) cells [30] . To determine whether E2-K233E also increases CHIKV fitness in A. albopictus , it was introduced into the SL07-226V background, and tested in competition experiment against SL07-226V_Apa. Surprisingly, the increase in CHIKV fitness due to the E2-K233E substitution was higher than that generated by any previously characterized second-step A. albopictus -adaptive mutation. No individual mosquitoes that ingested mixed competition blood meals exhibited a disseminated infection with only wt virus in the head, and wt RNA was present in mosquito body homogenates only in amounts that were insufficient for quantitative analysis ( Fig. 7l,p ). A 5.7-fold increase occurred in E2-K233E RNA over SL07-226V_Apa at 1 dpi ( Supplementary Fig. 7c ), which was similar to the effects of the E2-K210Q (fivefold) [18] and E2-K252Q (5.7-fold ( Fig. 5c )) substitutions. These findings suggest that, in addition to its effect on midgut infection, E2-K233E also increases CHIKV fitness in other mosquito organs/tissues. In addition to the E2-K233E substitution, the artificial E2-K234E substitution also resulted in a significant (one-tailed McNemar test, P <0.001) increase in fitness for infection of A. albopictus ( Fig. 7m,q ). Interestingly, introduction of E instead of the naturally occurring Q at position E2-252 also led to a significant increase (one-tailed McNemar test, P =0.026) in fitness in A. albopictus ( Fig. 7n,r ), indicating that amino acids Q and E are nearly interchangeable for this phenotype. Combined expression of E2-210Q and E2-252Q Identification of several second-step A. albopictus -adaptive mutations in the E2 gene raised the question of whether simultaneous expression of two or more such mutations might result in an additive or cooperative effect on CHIKV fitness, and thus could lead to selection of even more A. albopictus- transmissible strains in the future. To address this possibility, we combined substitutions E2-L210Q and E2-K252Q, which epidemiological data indicate circulate in India [11] and Southeast Asia, respectively ( Fig. 1 ). If there is an additive or cooperative effect between E2-L210Q and E2-K252Q, a ‘super-adapted’ strain could emerge in either location through simple Darwinian evolution. To test this hypothesis, we introduced mutations E2-L210Q and E2-K252Q into the SL07-226V_Apa background and tested the resulting double mutant (DM) virus in competition experiments against viruses expressing these individual E2 mutations. The results revealed 3.4- and 2.4-fold increases in the relative RNA amount ratio of DM compared with the E2-210Q and E2-252Q single-mutant competitors, respectively, in whole A. albopictus bodies assessed at 10 dpi ( Fig. 8 ). In addition, the DM was significantly more efficient (one-tailed McNemar test, P <0.05) in its ability to develop a disseminated infection represented by virus reaching A. albopictus heads, compared with either of the single-mutant competitors ( Fig. 8 ). This indicated that simultaneous expression of both second-step mutations led to an additive increase in CHIKV fitness. The fitness of the DM was also compared with the single mutants in 2-day-old mice. Although the RNA ratio of DM virus in mouse blood decreased slightly (1.5-fold) compared with either of the single-mutant competitors at 1 dpi, this ratio returned to almost 1.0 at 2 dpi ( Supplementary Fig. 8 ). These results indicate that the DM and single mutants have similar chances of being delivered orally to a mosquito via viremia. Overall, our data suggest that CHIKV-adaptive landscapes should favour the selection of a third-step A. albopictus -adaptive substitution in strains currently circulating in India and Southeast Asia. 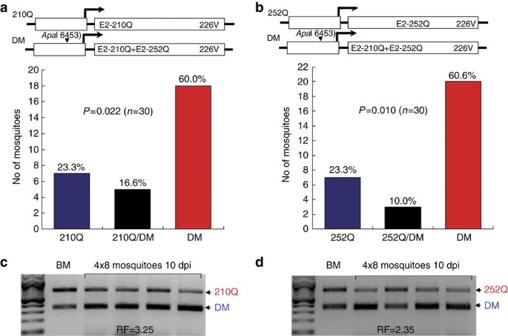Figure 8: Effect of combined expression of E2-L210Q and E2-K252Q on CHIKV fitness inA. albopictus. (a,b) above figures is a schematic representation of viruses used in the competition assay. Blood meals (BMs) containing 3 × 105p.f.u. ml−1of 1:1 mixture of viruses (DM and SL07-226V-210Q) (a,c) and (DM and SL07-226V-252Q) (b,d) were presented toA. albopictus. Disseminated CHIKV infection (a,b) and relative CHIKV RNA levels in mosquito bodies (c,d) were assayed at 10 dpi as described above. Graphs (a,b) show numbers and percent of mosquitoes containing DM, single mutant (SM; E2-L210Q or E2-K252Q), or containing both viruses in individual mosquito heads (representing disseminated infections). For each virus pair the difference in number of mosquitoes with disseminated infection of DM versus SM was tested for significance with a one-tailed McNemar test. Gel images (c,d) show change in relative RNA levels for each virus pair. RNA was extracted from BM at 0 dpi or 4 pools of 8 mosquitoes per pool at 10 dpi followed by RT-PCR analysis andApaI digestion to distinguish marked from unmarked competitors in amplicon gels. The relative fitness (RF) was determined as a geometric mean of the ratio between DM: SM amplicon bands in the sample, divided by the starting ratio of DM: SM bands in the BM. Figure 8: Effect of combined expression of E2-L210Q and E2-K252Q on CHIKV fitness in A. albopictus. ( a , b ) above figures is a schematic representation of viruses used in the competition assay. Blood meals (BMs) containing 3 × 10 5 p.f.u. ml −1 of 1:1 mixture of viruses (DM and SL07-226V-210Q) ( a , c ) and (DM and SL07-226V-252Q) (b,d) were presented to A. albopictus . Disseminated CHIKV infection ( a , b ) and relative CHIKV RNA levels in mosquito bodies ( c , d ) were assayed at 10 dpi as described above. Graphs ( a , b ) show numbers and percent of mosquitoes containing DM, single mutant (SM; E2-L210Q or E2-K252Q), or containing both viruses in individual mosquito heads (representing disseminated infections). For each virus pair the difference in number of mosquitoes with disseminated infection of DM versus SM was tested for significance with a one-tailed McNemar test. Gel images ( c , d ) show change in relative RNA levels for each virus pair. RNA was extracted from BM at 0 dpi or 4 pools of 8 mosquitoes per pool at 10 dpi followed by RT-PCR analysis and Apa I digestion to distinguish marked from unmarked competitors in amplicon gels. The relative fitness (RF) was determined as a geometric mean of the ratio between DM: SM amplicon bands in the sample, divided by the starting ratio of DM: SM bands in the BM. Full size image In this study, we demonstrated that acquisition of second-step A. albopictu s-adaptive mutations by CHIKV strains that already possess the first-step E1-A226V substitution has occurred on at least three separate occasions ( Figs 1 and 2 ). The detection of A. albopictus -adaptive mutations only in a subset of sl3 strains (clade sl3-B ) may reflect that the 2008 outbreak in Sri Lanka involving this clade was geographically confined during the initial phase of a selective sweep, restricting the propagation of the most fit viruses in a limited geographic range. Consistent with this explanation, CHIK cases were only reported in Sri Lanka from February and April, 2008 [11] , with no subsequent activity detected on the island. Another potential explanation is that one or more of these mutations had minor adaptive properties specific to certain geographic populations of mosquitoes that we did not test. More surprising are our findings showing that two independent A. albopictu s-adaptive substitutions (E2-L210Q and E2-K252Q) occurred in CHIKV strains circulating in the same location (Kerala, India) 2 years apart [25] , [31] . To our knowledge there is no evidence that sl4 strains from 2009 replaced via a selective sweep the Kerala 2007 ( sl1 ) strains. A more plausible explanation is that the E2-L210Q- and E2-K252Q-adaptive substitutions occurred independently during two separate outbreaks, each increasing transmission by A. albopictus compared with the parental strains with only the first-step E1-A226V-adaptive substitution [25] . Importantly, in subsequent years, both of these sub-lineages invaded Southeast Asia ( Fig. 1 ) [27] and northeastern India, conferring their evolutionary success. Our data demonstrate that, after CHIKV reached the first-step E1-A226V A. albopictu s-adaptive peak, its evolution was no longer constrained to a monolithic peak and multiple adaptive peaks of relatively equal fitness became available for Darwinian evolution. This finding challenges the traditional [20] , [32] two-step model of host switching adaptive evolution ( Fig. 9a ). Instead of forcing convergence of lineages into a single high-fitness peak by the acquisition of consecutive (first, second and third step and so on) adaptive mutations, the first-step E1-A226V adaptation permitted rapid lineage diversification ( Fig. 9b ) as different sets of secondary mutations provided similar, additional fitness gains. Although phylogenetic evidence indicates that the E1-A226V substitution preceded the signature substitutions in sl1 , sl3 and sl4 , our data do not indicate whether there was any dependence of the latter on the former. The order of acquisition may simply reflect the far stronger selective advantage of E1-A226V compared with the other substitutions [18] , which therefore would be expected to occur first during the evolution of CHIKV in regions inhabited by A. albopictus . 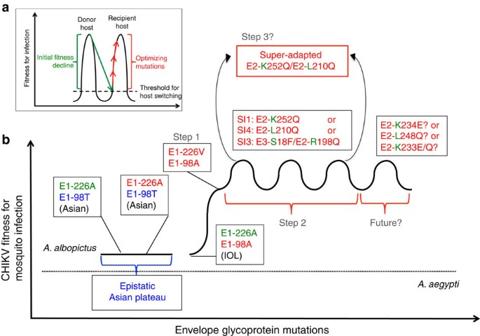Figure 9: Hypothetical and empirical fitness landscapes for a multi-step process of host switching by CHIKV. (a) The traditional hypothetical model20,32postulates an initial decline in fitness upon a host change due to the non-overlapping fitness landscapes, followed by gradual adaptive evolution to a single peak in a recipient host, which also results in a fitness decline for infection of the donor host. (b) Empirical model of CHIKV adaptation toA. albopictusshows the lack of an initial fitness decline upon shifting fromA. aegypti, and the existence of multiple, independent second-step adaptive peaks available after the initial adaptive E1-A226V substitution. Green indicates ancestral amino acids and red indicates derived. The Asian plateau represents the inability of Asian strains to reach the first-step adaptive peak owing to its dependence on the epistatic E1-A226V/E1-98T interaction (blue)2. Fitness forA. aegyptiinfection is not affected by any of theA. albopictus-adaptive substitutions. Figure 9: Hypothetical and empirical fitness landscapes for a multi-step process of host switching by CHIKV. ( a ) The traditional hypothetical model [20] , [32] postulates an initial decline in fitness upon a host change due to the non-overlapping fitness landscapes, followed by gradual adaptive evolution to a single peak in a recipient host, which also results in a fitness decline for infection of the donor host. ( b ) Empirical model of CHIKV adaptation to A. albopictus shows the lack of an initial fitness decline upon shifting from A. aegypti , and the existence of multiple, independent second-step adaptive peaks available after the initial adaptive E1-A226V substitution. Green indicates ancestral amino acids and red indicates derived. The Asian plateau represents the inability of Asian strains to reach the first-step adaptive peak owing to its dependence on the epistatic E1-A226V/E1-98T interaction (blue) [2] . Fitness for A. aegypti infection is not affected by any of the A. albopictus -adaptive substitutions. Full size image Our results also challenge traditional views of arbovirus evolution [30] , [33] , [34] in that specific adaptation to a given host (in this case A. albopictu s) was not accompanied by a major ‘trade-off’ of fitness for infection of alternate hosts ( A. aegypti or models for human infection), although some studies suggest a minor fitness reduction in this vector caused by E1-A226V [19] , [35] . A similar result was reported for a Venezuelan equine encephalitis virus mosquito ( A. taeniorhynchus )-adaptive substitution [36] , which also had no effect on infection of the original enzootic or donor vector, Culex ( Melanoconion ) taeniopus [37] . Overall, our findings somewhat mirror traditional Darwinian models of macroevolution, where major adaptations, such as development of wings by ancestors of birds, or the E1-A226V substitution in the case of CHIKV, can result in the rapid radiation/diversification of new lineages/species. The sl2 was the only CHIKV clade from Southeast Asia with the E1-A226V substitution for which we did not observe evidence for selection of second-step A. albopictu s-adaptive mutations. It is possible that such selection occurred at a stage of mosquito infection subsequent to dissemination into the haemocoel (for example, viral secretion to saliva by A. albopictu s salivary gland acinar cells), but was not detected by our method that only compared the ability of CHIKV to develop a disseminated infection, but not to establish transmission competence. Alternatively, sl2- specific mutations could have been acquired by this lineage as a result of CHIKV adaptation to alternative hosts, possibly humans. For instance, SL07-226V_Apa- sl2 was the only virus that exhibited increased fitness over SL07-226V (wt strain) in infant mice at early time points post infection (1 dpi) and in HFF cells, while viruses with sl1- and sl3 -specific mutations were both outcompeted by wt CHIKV in these surrogate models of human infection ( Figs 3 and 4 ). Interestingly, sl2 acquired the E1-K211N substitution convergently with strains of the old Asian CHIKV genotype that diverged from East Central South African ancestral genotype at least 60–70 years earlier than the IOL lineage [38] . Recently, we demonstrated that evolution of the Asian CHIKV genotype is epistatically constrained in its ability to adapt to A. albopictu s [2] , which indirectly supports the hypothesis that sl2 -specific second-step mutations were selected as a result of CHIKV adaptation to an alternative host. Finally, our data suggest that continued adaptation of IOL strains for transmission by A. albopictu s, owing to the accumulation of second- and possibly third-step mutations, may result in gradual displacement of the old Asian CHIKV lineage from A. albopictu s-abundant regions of Southeast Asia. The existences of latter lineage in nature should depend on its ability to invade and successfully compete with the IOL lineage in new geographic regions where A. albopictu s is not abundant. This scenario is consistent with recent CHIKV invasion of the Caribbean islands, where it is apparently transmitted primarily by A. aegypti [39] . The introduction of the Asian rather than the IOL lineage may have been stochastic, but our previous results [2] predict that these Caribbean strains will have a limited ability to adapt to A. albopictus , which may limit their spread into temperate regions of the Americas. This further underscores the need for understanding of the evolutionary mechanism that is involved in emergence of this major public health threat. Our approach of combining phylogenetic inference with experimental fitness evaluation of potential adaptive mutations in various hosts provides important insights into the molecular mechanisms of CHIKV evolution. All A. albopictu s-adaptive amino-acid substitutions we identified are located along or immediately adjacent to an axis formed between glutamine residues at E2 positions 210 and 252 ( Figs 2 and 7 ) [28] , and share the common effect of increasing initial infectivity/replication in A. albopictu s midgut cells ( Figs 5 and 6 ; Supplementary Fig. 7 ). The importance of this ‘axis of substitutions’ in the mechanism of adaptation was further supported by its ability to predict that the artificial E2-K233Q substitution would increase CHIKV fitness for infection of A. albopictu s to a level comparable to that generated by natural, adaptive mutations ( Fig. 7 ). In contrast, the second-site substitutions in sl2 , which did not show an adaptive advantage, are not located near this axis ( Fig. 2 ). The variation in effects among substitutions along this axis ( Fig. 7 ) most likely reflects the complexity of intermolecular protein–protein interactions within the CHIKV E3/E2/E1 spike. For instance, penetrance of the A. albopictu s-adaptive substitution E2-R198Q from sl3-B requires the additional E3-S18F substitution ( Fig. 2 ; Supplementary Fig. 6 ). E3 has been suggested to act as a clamp or brace holding E2 and E1 together during assembly [28] , [40] , [41] , [42] . Thus, E3-S18F may affect how the E2–E1 heterodimer containing E2-198Q is stabilized during assembly. The role of E3-S18F in the penetrance of E2-R198Q suggests that additional mutations may also be required for stabilizing glutamine residues at E2 positions 213, 232 and 248. Importantly, the positive effect of E2-K233Q on CHIKV fitness prompted investigation of the natural E2-K233E A. albopictu s-adaptive mutation, which was acquired by only one virus strain ( Fig. 1 ), and would not have been tested without the identification of the axis pattern. Our analysis showed that glutamine and glutamic acid residues at this position have similar effects on CHIKV fitness, and these residues also produce similar phenotypes at E2-252 ( Fig. 7 ; Supplementary Fig. 5 ). Together, our results demonstrate that the acquisition of either glutamine and/or glutamic acid at multiple positions along the E2-210-252 axis promotes the emergence of novel CHIKV sub-lineages characterized by increased fitness in A. albopictus. Thus, these findings will have important implications for future CHIKV surveillance to identify further adaptation to this important vector. The ‘axis of adaptive substitutions’ is located along the ASR of the E2 protein ( Supplementary Fig. 9 ) that connects domain B (the receptor-binding domain) with domains A and C and contacts both the E3 and E1 proteins through a network of hydrogen bonds and Van der Waals interactions [28] . Importantly, the ASR region is proposed to undergo a conformational change in response to receptor binding and the low-pH environment of the endosome during entry [28] , [40] , [43] , [44] . Previously, we hypothesized that the first-step E1-A226V substitution increases CHIKV fitness by sensing a favourable lipid composition for insertion of the E1 fusion loop into the target endosomal membrane [2] , [19] . Accordingly, the second-step adaptive mutations in the ASR may act by enhancing the effect of E1-A226V in regulating CHIKV fusion dynamics in endosomes of A. albopictu s by initiating a targeted, low-pH-induced E2–E1 heterodimer dissociation in the correct compartment, thereby improving fusion loop insertion. In this model, substitutions do not directly modify the receptor-binding site but rather their presence in the ASR may affect the course of entry, perhaps allowing fusion in the early rather than the late endosome. Alternatively, the second-step substitutions may simply increase CHIKV’s affinity for one or more receptors expressed on the apical surface of A. albopictus but not A. aegypti midgut epithelial cells, thus resulting in more efficient entry only in the former mosquito. An apparent trend in the evolution of the CHIKV IOL since its emergence in 2004 is its incremental, sequential increase in fitness for transmission by A. albopictus . Assuming that this vector remains important for transmission, its selection of even more transmissible strains should continue for the foreseeable future. Our results indicate that emergence of further adapted strains is likely because the artificial combination of two different second-step adaptive mutations yielded a CHIKV strain that was significantly more efficient (an approximate threefold increase, one-tailed McNemar test, P <0.05) in its ability to develop a disseminated infection in A. albopictus ( Fig. 8 ). These data demonstrate that current CHIKV strains have not yet reached a locally maximum adaptive peak for A. albopictus transmission, and suggest that individual second-step adaptive peaks possess the potential for convergence into a single or multiple ‘super-adaptive’ peaks in the future in at least two endemic locations ( Fig. 9b ). Although our results suggest that further adaptation to A. albopictus will not result in major tradeoffs of reduced fitness in A. aegypti or human hosts, the limited fidelity of rodents to model human infections limits our ability to estimate CHIKV fitness for human viremia. Thus, our observation of a slight (~1.5-fold) decrease in replication of the DM compared with single-mutant viruses in infant mice at 1 dpi ( Supplementary Fig. 8 ) should be corroborated by infections of nonhuman primates that more accurately reflect human infection [45] . If a slight decrease in human viremia potential accompanies the combination of second-step A. albopictus -adaptive mutations, they may not be efficiently selected in nature. In conclusion, we demonstrated that the initial E1-A226V A. albopictus -adaptive CHIKV substitution has been followed by several second-step, adaptive mutations in its envelope glycoprotein genes that further increased CHIKV fitness in this mosquito vector. Surprisingly, these species-specific adaptations do not have major effects on infection of the alternate urban mosquito vector, A. aegypti , or models for human infection. These findings challenge the trade-off hypothesis for arbovirus evolution, which predicts that most adaptive arbovirus mutations will be deleterious in donor or alternate hosts. Finally, our findings indicate that even more efficient CHIKV transmission by the invasive vector A. albopictus will likely evolve when combinations of these second-step mutations occur in their current ranges of endemic circulation in India and Southeast Asia, followed by their likely global spread. Viruses and plasmids The E1-A226V derivative of an infectious cDNA clone (i.c.) of the SL07 (SL-CK1) CHIKV strain with and without an Apa I marker (SL07-226V and SL07-226V_Apa) have been described previously [2] , [18] . SL07 was isolated from a febrile patient in Sri Lanka in 2007 (GenBank accession number HM045801.1 ), and was passed two times on Vero cells before i.c. construction. The Thailand-2009_CK11/53 strain was isolated from human serum collected on 16 September 2009. Serum was used for infection of confluent monolayers of C6/36 cells. Supernatant was harvested 2 days post infection (dpi), aliquoted and stored at −80 °C before being used for sequencing and/or competition experiments. For genome sequencing, viral RNA was extracted from C6/36 cells supernatants using TRIzol reagent (Invitrogen, Carlsbad, CA), reverse-transcribed using Superscript III (Invitrogen) and cDNA was amplified using Taq DNA polymerase (New England Biolabs (NEB), Ipswich, MA). PCR fragments were purified from 1% agarose gel using the Zymoclean Gel DNA Recovery Kit (Zymo Research, Irvine, CA) and sequenced using 3500 Genetic Analyzer (Applied Biosystems, Foster City, CA) according to manufacturer’s instructions. All point mutations of interest were introduced individually or in various combinations into the i.c. of SL07-226V_Apa and SL-226V using PCR-based techniques [46] followed by swapping of gene segments using conventional cloning methods [46] . The PCR-generated regions and regions of genetic swaps were completely sequenced to validate genetic integrity of the constructs. Plasmids were propagated using the TOP10 strain of E. coli (Invitrogen) in Terrific Broth medium followed by purification using the cesium chloride gradient centrifugation method. Detailed information for all plasmids is available from the authors on request. Cells and mosquitoes Vero cells (African green monkey kidney) were maintained at 37 °C, with 5% CO 2 , in minimal essential medium (MEM; Invitrogen) supplemented with 5% fetal bovine serum (FBS), and 1 × penicillin/streptomycin solution. Primary HFFs (ATCC, CRL-2522) were maintained in Dulbecco’s MEM (Invitrogen) supplemented with 10% FBS, 1 × penicillin/streptomycin, 2 mM L -glutamine and 1 × nonessential amino-acids solution (Sigma-Aldrich, St Louis, MO). C6/36 cells ( A. albopictus ) were maintained in MEM-alpha (Invitrogen) supplemented with 10% FBS and 1 × vitamin solution. Galveston and Thailand colonies of A. albopictus and a white-eyed Higgs variant of the Rexville D strain of A. aegypti mosquitoes have been described earlier [2] , [47] , [48] , [49] . All manipulations and handling of mosquitoes were done as described previously [50] . Recovery of the infectious viruses To minimize variability between viruses to be compared in competition experiments, all rescuing procedures were performed simultaneously. Infectious viruses were generated by electroporation of in vitro -transcribed RNA into Vero cells as described previously [18] . Plasmids were linearized with Not I restriction endonuclease (NEB), followed by phenol–chloroform purification. A 5′-capped virus RNA was in vitro transcribed from SP6 promoter located upstream of the viral genome using the mMESSAGE mMACHINE kit (Ambion, Austin, TX). RNA was transfected in 4-mm cuvettes into 10 7 Vero cells by electroporation using a BTX-Harvard Apparatus ECM 830 Square Wave Electroporator (Harvard Apparatus, Holliston, MA) and the following conditions: 250 V, pulse length 10 ms, 3 pulses, with an interval between the pulses of 1 s. Cells were suspended in 14 ml of Leibovitz L-15 (L-15) medium supplemented with 10% FBS and 5% tryptose phosphate broth (Sigma-Aldrich) and allowed to attach to a 75-cm 2 flasks for 3 h. The medium was replaced with 14 ml of L-15 and maintained at 37 °C without CO 2 . To monitor virus recovery, samples were collected at 24 and 48 h and stored at −80 °C. The specific infectivity of electroporated RNAs was assessed as described previously [18] . An aliquot containing 1/100 of electroporated Vero cells (1 × 10 5 ) was serially 10-fold diluted and seeded on sub-confluent monolayers (1 × 10 6 cells per well) of uninfected Vero cells in six-well plates, then incubated for 2 h at 37 °C [47] . Plaques were developed by incubation of the plates at 37 °C for 48 h overlaid with 0.5% agarose in MEM supplemented with 3.3% FBS. The specific infectivity values were expressed as plaque-forming unit (p.f.u.) per microgram of electroporated RNA ( Supplementary Tables 1–5 ). Titres of the viruses after electroporation were determined by titration on Vero cells by plaque assay as previously described [51] . Mosquito infections Comparison for the effect of mutations of interest on CHIKV dissemination in A. albopictus and A. aegypti mosquitoes was performed using a direct competition experiment as described earlier [2] , [19] . A pair of viruses that differed by mutations of interest was mixed at a 1:1 ratio (based on p.f.u. ), with one of the viruses containing the Apa I marker. The resulting mixes were further diluted depending on the experiment to: 6 × 10 5 , 2 × 10 6 or 2 × 10 7 p.f.u. ml −1 with L-15 medium. Infectious blood meals were prepared by dilution of virus in an equal volume of the defibrinated sheep blood (Colorado Serum, Denver, CO), then orally presented to 100 4 to 5-day-old female mosquitoes using a Hemotek membrane feeding system (Discovery Workshops, Accrington, Lancashire, UK) as described previously [19] , [50] . At 7 or 10 dpi, heads of individual mosquitoes were triturated in 500 μl of MEM media containing 5 μg ml −1 of Amphotericin B (Fungizone (Sigma-Aldrich)). Supernatants were clarified by centrifugation at 16,000 g and 100 μl of media were used for infection of 5 × 10 4 Vero cells per well in duplicates in 96-well plates. Plates were incubated for 72 h at 37 °C, to allow the virus-induced cytopathic effect to develop. Supernatants from cytopathic effect-positive wells were used for RNA extraction followed by RT–PCR amplification of the Apa I containing CHIKV genome region with 41855ns-F5 (5′-ATATCTAGACATGGTGGAC-3′) and 41855ns-R1 (5′-TATCAAAGGAGGCTATGTC-3′) primers using the One-Step RT–PCR kit (Qiagen, Valencia, CA). The PCR products were digested with a mix of Apa I and PspOM I restrictases (NEB) and separated on 1.5% agarose gels followed by ethidium bromide staining. One PCR band in the digested sample corresponded to disseminated infection for one out of two viruses in the pair; two bands indicated that both viruses have developed disseminated infection in the same mosquito. Differences in dissemination efficiencies between two competitors were tested for significance with a one-tailed McNemar test. To evaluate the effects of mutations of interest on accumulation of CHIKV RNA in whole mosquito bodies or midguts, mosquitoes were exposed to blood meals containing 1:1 mixes of viruses that differed by a set of mutations of interest as described above. At 1, 2 and 3 dpi, mosquito midguts were collected in pools of 10, in duplicate, and were used for RNA extraction using TRIzol reagent. For whole mosquitoes, total RNA was extracted from pools of 10 mosquito bodies in quadruplicate at 7 or 10 dpi. RNA was RT-PCR amplified, followed by Apa I and PspOM I digestion of amplicons as described above. Gel images were analysed using TolaLab (version 2.01, TolaLab LTD) and relative fitness for a given virus pair during competition was determined as the ratio between Apa I marked and unmarked virus RNA in the sample, and their starting ratio in the blood meal. The results were expressed as a geometric mean of relative fitness for 2 pools of 10 mosquito midguts, or 4 pools of 10 mosquito bodies. The images for the full gels are provided in Supplementary Materials ; ( Supplementary Figs 10–14 ). Competition assays in Vero and HFF cells To investigate the effect of mutations of interest on CHIKV fitness in Vero and HFF cells, the cells were grown to 95% confluence in a six-well plate and infected in triplicate with 1:1 mixes of the corresponding viruses at an MOI of 0.1 p.f.u. per cell for 1 h at 37 °C. Cells monolayers were washed three times with MEM-alpha, followed by incubation at 37 °C with 5% CO 2 . Cell culture supernatants were collected at 1 and 2 dpi, and used for RNA extraction followed by RT-PCR analysis as described above. The images for the full gels are provided in Supplementary Materials ; ( Supplementary Fig. 15 ). Competition assays in mice All animal manipulations were approved by the University of Texas Medical Branch Institutional Animal Care and Use Committee and conformed to the Association for Assessment and Accreditation of Laboratory Animal Care standards. To evaluate the effect of mutations of interest on CHIKV fitness in infant mice, a pair of viruses that differed by mutations of interest was mixed at a 1:1 ratio and diluted to 2 × 10 3 p.f.u. ml −1 with PBS/2% FBS. A litter of 2 to 3-day-old CD1mice (Charles River, Wilmington, MA) were subcutaneously infected with 50 μl of CHIKV mixes (10 2 p.f.u. per mouse). Blood from individual animals killed on day 1 or 2 post exposure was used for total RNA extraction with TRIzol reagent. The RNA was processed as described above. The results were expressed as a geometric mean of relative fitness values for analysed competitors from 4–5 individual mice. The images for the full gels are provided in Supplementary Materials ; ( Supplementary Fig. 16 ). Phylogenetic and selection pressure studies All available complete genome sequences representing the Indian Ocean Epidemic (IOL) lineage, along with an outgroup strain (Indian/MH4/2000) from ECSA lineage were downloaded from GenBank ( Supplementary Table 7 ). Additional sequences of IOL strains from a Kerala outbreak 2009 and Thailand outbreak 2008–2009 were generated by sequencing of viruses recovered from patient serum ( Supplementary Table 7 ). In total, 91 CHIKV whole-genome sequences were used for this analysis. Sequence alignment was performed first using MUSCLE [52] , followed by manual adjustment in Se-Al (available at http://tree.bio.ed.ac.uk/software/seal/ ) to preserve codon homology. Highly diverged 3′-untranslated regions and other rapidly evolving untranslated regions were excluded from analysis owing to the ambiguous alignment and/or ‘multiple hits’ problems that hinder accuracy. Only open-reading frames were adopted in further analysis. This led to an alignment length of 11,163 nt. Phylogenetic relationships of the 91 representative strains was reconstructed via the maximum likelihood method implemented in PAUP* v4.0b [53] , utilizing the best-fit model estimated using MODELTEST [54] . The robustness of each node was estimated using bootstrap resampling (1,000 replications) under the neighbor-joining procedure, with input genetic distances determined under the ML substitution model. The amino-acid changes along the branches were traced using MacClade 4 software [55] . Positively selected codon sites in the CHIKV genome were estimated by the internal fixed-effects likelihood method using HYPHY package [56] . This method only accounts for substitutions along internal branches, therefore is more suitable for selection pressure estimation at population level, where external transient mutations will not be fixed [57] . Accession codes: DNA sequences generated in this study have been deposited in GenBank nucleotide database under the accession codes KJ796844 to KJ796852 . How to cite this article : Tsetsarkin, K. A. et al. Multi-peaked adaptive landscape for chikungunya virus evolution predicts continued fitness optimization in Aedes albopictu s mosquitoes. Nat. Commun. 5:4084 doi: 10.1038/ncomms5084 (2014).